Thyroid hormone determines the start of the sensitive period of imprinting and primes later learning Filial imprinting in precocial birds is the process of forming a social attachment during a sensitive or critical period, restricted to the first few days after hatching. Imprinting is considered to be part of early learning to aid the survival of juveniles by securing maternal care. Here we show that the thyroid hormone 3,5,3′-triiodothyronine (T 3 ) determines the start of the sensitive period. Imprinting training in chicks causes rapid inflow of T 3 , converted from circulating plasma thyroxine by Dio2, type 2 iodothyronine deiodinase, in brain vascular endothelial cells. The T 3 thus initiates and extends the sensitive period to last more than 1 week via non-genomic mechanisms and primes subsequent learning. Even in non-imprinted chicks whose sensitive period has ended, exogenous T 3 enables imprinting. Our findings indicate that T 3 determines the start of the sensitive period for imprinting and has a critical role in later learning. Filial imprinting in precocial birds has been studied intensively [1] , [2] , [3] . Newly hatched chicks and ducklings follow the first conspicuous moving object they see. This is the biological mother under normal conditions. However, under experimental conditions it can, in theory, be any other object. While following, the birds learn the colour and shape of the object and become attached to it [4] . This learning behaviour, called filial imprinting, is restricted to a sensitive period [5] that lasts only a few days in the case of chicks and ducklings. There are several theories concerning the control of the time course of this sensitive period [6] , [7] , [8] , [9] , about which very little was known, including the existence of a determining factor [10] , [11] , [12] . Filial imprinting in nature consists of visual and auditory stimuli. The intermediate medial mesopallium (IMM, an association area of the telencephalon) in chicks ( Gallus gallus domesticus ) has a critical role in visual imprinting [2] , [13] , [14] . Bilateral ablation of the IMM prevents imprinting and abolishes the acquisition of filial preferences [13] . Electron microscopic studies show that the morphology of synapses in the IMM is modified by imprinting [15] . In addition, total RNA synthesis is upregulated in the IMM during the acquisition phase of imprinting [16] , suggesting that gene expression in the IMM is involved in the process of imprinting. Another brain region, the medio-rostral nidopallium/mesopallium (MNM) has been identified as the auditory-imprinting-relevant region [17] , [18] and its involvement of the MNM in sexual imprinting was confirmed in zebra finches [19] . Thus, taking the works on visual and auditory imprinting together, it seems likely that a broad network of connected forebrain regions, including the IMM, MNM and other forebrain regions, work together during imprinting and memory formation. We previously determined the genes that are preferentially expressed in the IMM of the brains of imprinted chicks 6 h after initiation of imprinting training [20] , [21] , but the molecular mechanism that regulates the sensitive period of imprinting was not clarified. Here we present results indicating the involvement of the thyroid hormone 3,5,3′-triiodothyronine (T 3 ), in controlling the timing of the sensitive period. We find that imprinting causes rapid inflow of thyroid hormone in chick brain through enhanced conversion by Dio2, type 2 iodothyronine deiodinase, in the endothelial cells of brain capillaries, enabling imprinting specifically via non-genomic mechanisms. The data from our experiments indicate that thyroid hormone in chick brain is a determining factor for the sensitive period of imprinting. This hormone can reopen a previously closed sensitive period and enable imprinting again. It can also confer what we term 'memory priming (MP)' to prime later learning. Once chicks have achieved memory priming, it is maintained for long periods, for over 1 week. This study elucidates the critical role of imprinting to subsequent learning as being governed by the acute action of thyroid hormone. Dio2 is upregulated in brain capillaries following imprinting We attempted to identify the genes differentially expressed at an earlier phase of imprinting than reported previously [20] . One-day-old chicks were trained for imprinting for 1 h and whole brains were collected and used for complementary DNA microarray and quantitative reverse transcription–polymerase chain reaction. We identified 18 genes, including Dio2, Type 2 iodothyronine deiodinase, that upregulated accompanying imprinting ( Fig. 1a ; Supplementary Tables S1 and S2 ). We focused on Dio2, the enzyme that catalyses the intracellular deiodination of thyroxine (T 4 ) prohormone to the active T 3 , because the concentrations of thyroid hormones in plasma were reported to peak around hatching in precocial birds [22] . Thyroid hormone is synthesized as T 4 in thyroid, circulates in blood vessels and reaches the endothelial cells of brain capillaries [23] . Using in situ hybridization, mRNA for Dio2 was found to be ubiquitously accumulated in the imprinted chicks' brains, including the IMM, and its expression was enriched in brain capillaries ( Fig. 1b–h ). Immunohistochemistry showed that Dio2 co-localized with P-glycoprotein, a marker of brain capillaries ( Fig. 1i–k ), western blotting showed that Dio2 was fractionated in the capillary fraction ( Fig. 1l ) and Dio2 was recognized as a single band using anti-Dio2 antibody in the whole brain lysate ( Supplementary Fig. S1 ). Dio2 was also enriched in brain capillaries of the MNM, which has been identified as the auditory-imprinting-relevant region [17] , [18] , suggesting that visual imprinting may have some influence on the auditory-imprinting-relevant region ( Fig. 1m–p ). These results imply that Dio2 converts T 4 to T 3 in endothelial cells of brain capillaries and provides T 3 to brain cells for imprinting. 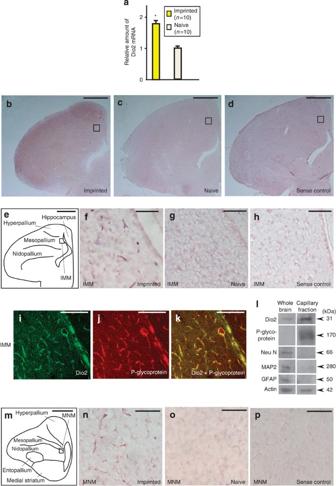Figure 1: Dio2 is upregulated in brain capillaries following imprinting. (a) Quantitative reverse transcription–polymerase chain reaction showed upregulation of Dio2 associated with imprinting. Mean±s.e.m. (U-test, *P<0.05). The numbers of animals used are indicated in parentheses. (b–d)In situhybridization showed Dio2 was upregulated ubiquitously in brains, including the IMM. (b,c) Antisense probe for Dio2 was used (b, imprinted;c, dark-reared). (d) Sense probe as a negative control was used. (e) Diagram of coronal section of left brain hemisphere. (f–h) High magnification of IMM (boxes). Dio2 was upregulated in brain capillaries associated with imprinting. (i–k) Dio2 protein was co-localized with P-glycoprotein. (i,j) Labelling of Dio2 protein (i) and P-glycoprotein (j), a marker for brain capillaries in the same section. (k) Images ofiandjhave been combined. (l) Immunoblotting showed that Dio2 was enriched in the capillary fraction. (m–p)In situhybridization showed that Dio2 was upregulated in brain capillaries associated with imprinting in the MNM. (m) Diagram of coronal section of the left brain hemisphere. (n–p) High magnification of MNM (box). (n,o) Antisense probes for Dio2 were used. (p) Sense probe as a negative control was used. (b–e,m) Scale bars, 2 mm. (f–k,n–p) Scale bar, 200 μm. GFAP, glial fibrillary acidic protein ; MAP, Microtubule-associated protein. Figure 1: Dio2 is upregulated in brain capillaries following imprinting. ( a ) Quantitative reverse transcription–polymerase chain reaction showed upregulation of Dio2 associated with imprinting. Mean±s.e.m. ( U -test, * P <0.05). The numbers of animals used are indicated in parentheses. ( b – d ) In situ hybridization showed Dio2 was upregulated ubiquitously in brains, including the IMM. ( b , c ) Antisense probe for Dio2 was used ( b , imprinted; c , dark-reared). ( d ) Sense probe as a negative control was used. ( e ) Diagram of coronal section of left brain hemisphere. ( f – h ) High magnification of IMM (boxes). Dio2 was upregulated in brain capillaries associated with imprinting. ( i – k ) Dio2 protein was co-localized with P-glycoprotein. ( i , j ) Labelling of Dio2 protein ( i ) and P-glycoprotein ( j ), a marker for brain capillaries in the same section. ( k ) Images of i and j have been combined. ( l ) Immunoblotting showed that Dio2 was enriched in the capillary fraction. ( m – p ) In situ hybridization showed that Dio2 was upregulated in brain capillaries associated with imprinting in the MNM. ( m ) Diagram of coronal section of the left brain hemisphere. ( n – p ) High magnification of MNM (box). ( n , o ) Antisense probes for Dio2 were used. ( p ) Sense probe as a negative control was used. ( b – e , m ) Scale bars, 2 mm. ( f – k , n – p ) Scale bar, 200 μm. GFAP, glial fibrillary acidic protein ; MAP, Microtubule-associated protein. Full size image Thyroid hormone signalling is involved in imprinting Indeed, intravenous injection of Dio2 inhibitors, iopanoic acid (IOP) and phloretin, impaired visual imprinting ( Fig. 2a–c ). To confirm the conversion from T 4 to T 3 by Dio2, we injected 125 I-labelled T 4 intravenously to detect 125 I-labelled T 3 converted from 125 I-labelled T 4 in brains. As a result, 125 I-labelled T 3 was detected mostly in the brain ( Fig. 2d ). Furthermore, intravenous injection of IOP reduced the amount of 125 I-labelled T 3 in brain ( Fig. 2e ), indicating that Dio2 did convert T 4 to T 3 in chick brains. Thus, it may be concluded that Dio2 converts T 4 to T 3 in endothelial cells of brain capillaries, providing T 3 to brain cells for imprinting. The IMM in chicks has a critical role in visual imprinting [2] , [13] , [14] . As shown in Fig. 2f,g , bilateral ablation of the IMM prevented imprinting, and abolished the acquisition of filial preferences as reported previously [13] . The converted T 3 in endothelial cells is assumed to be transported by a monocarboxylate transporter towards brain cells, incorporated in the cytoplasm and binds to thyroid hormone receptors (TRs) whose gene expressions were detected in the IMM ( Supplementary Fig. S2 ). In fact, imprinting was impaired by IMM injection with inhibitors of thyroid hormone signalling molecules (IOP; a monocarboxylate transporter 8 inhibitor, BSP; a thyroid hormone receptor antagonist, NH-3 (ref. 24 )), suggesting that accumulation of T 3 in the IMM of chick brain by thyroid hormone signalling in the blood–brain barrier is important for imprinting ( Fig. 2h ). As the TRs are reported to distribute in neuronal and glial cells in mammals [25] , T 3 probably affects neuron and/or glia through its receptor in chick. As Dio2 is upregulated in broad areas of chick brain including the IMM and MNM, thyroid hormone may be involved in a variety of brain functions around the time of hatching. Northern blotting showed Dio2 expression to be stronger in the brain and lung than in the liver, testis, thymus and skin ( Supplementary Fig. S3 ). In brains, Dio2 mRNA gradually accumulated from 3 days before hatching, peaked around hatching then leveled off and remained in steady state until 5 days after hatching ( Supplementary Fig. S4 ). As Dio2 is known to be induced by infectious stress in the brain [26] , Dio2 in other parts of the brain may be involved in the immune response against microorganisms under new circumstances after hatching. However, Dio2 upregulation by imprinting training is learning-dependent, but not infection-dependent, because the chicks reared as the control group in light-exposed condition without imprinting training did not show Dio2 upregulation. Another possibility is that the function of Dio2 in the neuronal network of other areas may be linked with the molecular events in the IMM and MNM, which would be necessary for the acquisition of imprinting behaviour. 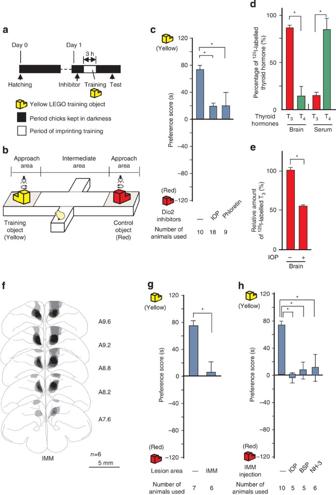Figure 2: Thyroid hormone signalling is involved in imprinting. (a) The schemes to test the effect of inhibitors for imprinting. Imprinting training and simultaneous choice test were carried out by the method of Izawaet al.44with modification (see detailed information in the Methods section). After hatching, chicks were kept in dark enclosures to prevent exposure to light until day 1. Then chicks were trained with a yellow LEGO object, and the preference for the yellow LEGO object was evaluated 1 h later. Imprinting training was initiated 30 min after the inhibitor injection. (b) Preference score was measured by the difference in approach time during 120 s; the time chicks spent near the control object (red) was subtracted from that chicks spent near the training object (yellow). Chicks stayed in each approach area or in the intermediate areas between the two areas during simultaneous choice test. Side walls on the alley and the arms are not drawn in this figure. (c) Imprinting was impaired by intravenous injection of Dio2 inhibitors (IOP and phloretin). (d,e) Converted T3flowed in brain. (d) Intravenously injected125I-labelled T4was detected mostly as T3in brains, but as T4in serum (n=4). (e) Amount of125I-labelled T3detected in brains was reduced by IOP (n=4). (f,g) IMM is required for imprinting on day 1. Ibotenic acid lesions were performed on day 0 and chicks were trained and tested on day 1. Training and testing for the preference followed the experimental scheme shown ina,b. (f) Histological reconstruction of ibotenic acid lesions in IMM. The lesioned areas are superimposed over coronal sections of telencephalon. (g) Effects of bilateral lesions of IMM on the acquisition of imprinting on day 1. (h) Imprinting was impaired by the IMM injection of inhibitors (Dio2 inhibitor, IOP; a monocarboxylate transporter 8 inhibitor, BSP; a thyroid hormone receptor antagonist, NH-3). Training and testing for preference followed the experimental scheme shown ina,b. (c,h) Mean±s.e.m. (Kruskal–Wallis test and subsequent multiple comparisons, *P<0.05). (d,e,g) Mean±s.e.m. (U-test, *P<0.05). The numbers of animals used are indicated in each figure (c,g,h). Figure 2: Thyroid hormone signalling is involved in imprinting. ( a ) The schemes to test the effect of inhibitors for imprinting. Imprinting training and simultaneous choice test were carried out by the method of Izawa et al . [44] with modification (see detailed information in the Methods section). After hatching, chicks were kept in dark enclosures to prevent exposure to light until day 1. Then chicks were trained with a yellow LEGO object, and the preference for the yellow LEGO object was evaluated 1 h later. Imprinting training was initiated 30 min after the inhibitor injection. ( b ) Preference score was measured by the difference in approach time during 120 s; the time chicks spent near the control object (red) was subtracted from that chicks spent near the training object (yellow). Chicks stayed in each approach area or in the intermediate areas between the two areas during simultaneous choice test. Side walls on the alley and the arms are not drawn in this figure. ( c ) Imprinting was impaired by intravenous injection of Dio2 inhibitors (IOP and phloretin). ( d , e ) Converted T 3 flowed in brain. ( d ) Intravenously injected 125 I-labelled T 4 was detected mostly as T 3 in brains, but as T 4 in serum ( n =4). ( e ) Amount of 125 I-labelled T 3 detected in brains was reduced by IOP ( n =4). ( f , g ) IMM is required for imprinting on day 1. Ibotenic acid lesions were performed on day 0 and chicks were trained and tested on day 1. Training and testing for the preference followed the experimental scheme shown in a , b . ( f ) Histological reconstruction of ibotenic acid lesions in IMM. The lesioned areas are superimposed over coronal sections of telencephalon. ( g ) Effects of bilateral lesions of IMM on the acquisition of imprinting on day 1. ( h ) Imprinting was impaired by the IMM injection of inhibitors (Dio2 inhibitor, IOP; a monocarboxylate transporter 8 inhibitor, BSP; a thyroid hormone receptor antagonist, NH-3). Training and testing for preference followed the experimental scheme shown in a , b . ( c , h ) Mean±s.e.m. (Kruskal–Wallis test and subsequent multiple comparisons, * P <0.05). ( d , e , g ) Mean±s.e.m. ( U -test, * P <0.05). The numbers of animals used are indicated in each figure ( c , g , h ). Full size image Thyroid hormones are critical factors for imprinting The concentration of thyroid hormones in brain and serum during development was determined using embryos and chicks. In brains, T 3 gradually accumulated from 6 days before hatching, peaked around hatching then decreased to background level 5 days after hatching, while T 4 became almost undetectable ( Fig. 3a ). In serum, concentrations of both T 3 and T 4 peaked around hatching ( Fig. 3b ). Also, the amount of T 3 in imprinted chicks was 1.7-fold higher than in dark-reared chicks, IOP-injected chicks or light-exposed control chicks kept in a training chamber where light was turned on and off but with no training object ( Fig. 3c ). No significant difference was found in serum thyroid hormones in these animals ( Fig. 3d ). The preference score in the test of imprinting was positively correlated with T 3 in brain, the amount of T 3 in good learners being higher than in poor learners ( Fig. 3e ). In this experiment, the time of the training session was shortened so a weak training protocol was used to yield good or poor learners. Because IOP injection impaired imprinting, as shown in Fig. 2c,h , a further increase in T 3 converted by Dio2 in the process of training was likely to be required for imprinting. We then examined whether thyroid hormones are determinants in imprinting. When T 3 was intravenously injected to 1-day-old chicks, chicks' preference was facilitated and not affected by IOP. Such facilitation was also found for T 4 , but the chicks' preference greatly decreased in the presence of IOP, suggesting that brain T 3 converted from T 4 by Dio2 is the determinant for imprinting ( Fig. 3f ). 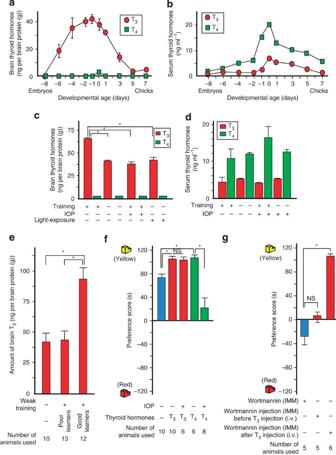Figure 3: Thyroid hormones are critical factors for imprinting. (a,b) Amount of thyroid hormones in brains (n=4,a) and in serum (n=4,b) during development. (c) Amount of thyroid hormones increased in brains by imprinting, but not in serum (d). (e) The amount of T3in good learners (n=12) was higher than in poor learners (n=13). Preference for the training object (yellow) was evaluated in the same way as shown inFig. 2b. In this experiment, the time of the training session was shortened so a weak training protocol was used to yield good or poor learners. The preference scores in the simultaneous choice test (during 120 s) of the good learners were over 80 s in the test for imprinting, and those of the poor learners were under 40 s. (f) Intravenous injection of thyroid hormones facilitated imprinting on day 1. (g) Effect of wortmannin on imprinting of 1-day-old chicks. (c–g) Mean±s.e.m. (Kruskal–Wallis test and subsequent multiple comparisons, *P<0.05). (c,d,f,g) The training, testing and injection were performed following the experimental scheme shown inFig. 2a. (e,f,g) The preference for the training object (yellow) was evaluated in the same way as shown inFig. 2b. The numbers of animals used are indicated in each figure (e–g). NS, nonsignificant. Figure 3: Thyroid hormones are critical factors for imprinting. ( a , b ) Amount of thyroid hormones in brains ( n =4, a ) and in serum ( n =4, b ) during development. ( c ) Amount of thyroid hormones increased in brains by imprinting, but not in serum ( d ). ( e ) The amount of T 3 in good learners ( n =12) was higher than in poor learners ( n =13). Preference for the training object (yellow) was evaluated in the same way as shown in Fig. 2b . In this experiment, the time of the training session was shortened so a weak training protocol was used to yield good or poor learners. The preference scores in the simultaneous choice test (during 120 s) of the good learners were over 80 s in the test for imprinting, and those of the poor learners were under 40 s. ( f ) Intravenous injection of thyroid hormones facilitated imprinting on day 1. ( g ) Effect of wortmannin on imprinting of 1-day-old chicks. ( c – g ) Mean±s.e.m. (Kruskal–Wallis test and subsequent multiple comparisons, * P <0.05). ( c , d , f , g ) The training, testing and injection were performed following the experimental scheme shown in Fig. 2a . ( e , f , g ) The preference for the training object (yellow) was evaluated in the same way as shown in Fig. 2b . The numbers of animals used are indicated in each figure ( e – g ). NS, nonsignificant. Full size image We next examined the mode of action of T 3 in the imprinting process. T 3 deficiency during brain development is associated with neurological disorder [27] through genomic action [23] . The non-genomic action of T 3 has also been described [28] . For example, the PI 3 Kinase/Akt pathway was reported to mediate the rapid non-genomic cardiovascular effects of TR [29] . Because injected T 3 affects imprinting rapidly within 30 min, it probably functions via a non-genomic action. We injected wortmannin, a PI 3 Kinase inhibitor, into the IMM to examine its effect on imprinting. Wortmannin injection 30 min before intravenous injection of T 3 hampered the effect of T 3 . However, wortmannin injected 30 min after T 3 treatment did not, indicating that the rapid non-genomic action of T 3 before the training contributed to imprinting ( Fig. 3g ). T 3 acts as a determinant for the sensitive period As increase in T 3 facilitated chicks' preference on day 1, we investigated whether increase in T 3 could affect the sensitive period of imprinting. We found that the sensitive period for imprinting was restricted to the first 3 days after hatching and that the period closed at day 4 when dark-reared chicks could no longer be imprinted ( Fig. 4a,b ). However, the dark-reared chicks injected with T 3 intravenously 30 min before the imprinting training showed strong preference on day 4 or day 6, showing that thyroid hormone acts as the determinant of the opening of the sensitive period ( Fig. 4b ; Supplementary Movie 1 ). The effect of T 3 on the acquisition of imprinting on day 4 was also shown using a running wheel apparatus [30] , which is different from the apparatus equipped with a computer-controlled rubber belt and the infrared sensor used in other experiments ( Supplementary Fig. S5 ). The injection of thyroid hormones and various inhibitors affected the acquisition of memory itself but not the locomotor activity of chicks ( Supplementary Fig. S6 ). However, on day 8 or day 10, thyroid hormones did not effectively enhance the preference of chicks, suggesting the presence of unidentified factors, which may contribute to the closing of the sensitive period ( Fig. 4b ). The effect of thyroid hormones on establishing chicks' preference on day 4 was dose-dependent ( Fig. 4c,d ), and the effective concentrations were consistent with those detected in 1-day-old chicks. These results indicate that a simple hormone, T 3 , may regulate the beginning of the sensitive period in imprinting. 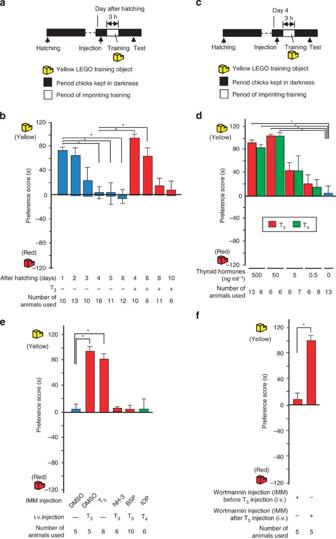Figure 4: T3acts as a determinant for the sensitive period. (a) The scheme for testing the effect of thyroid hormones for imprinting. (b) Dark-reared chicks were trained for imprinting with a yellow LEGO object and subsequently the preference for the yellow LEGO object was evaluated on a single day after hatching (from day 1 to day 10). The sensitive period closed on day 4 and chicks were not imprinted, whereas chicks injected with T330 min before the training became imprintable from day 4 to day 6. (c) The scheme for testing the effect of thyroid hormones on 4-day-old chicks ind–f. Dark-reared chicks were trained for imprinting with a yellow LEGO object and the preference for the yellow LEGO object was evaluated on day 4 after hatching in the same way as shown inFig. 2b. (d) Dose-dependent effects of thyroid hormones on 4-day-old chicks. (e) IMM injection of inhibitors (a thyroid hormone receptor antagonist, NH-3; a monocarboxylate transporter 8 inhibitor, BSP; Dio2 inhibitor, IOP) hampered the effect of thyroid hormones on 4-day-old chicks. (f) Effect of wortmannin on imprinting of 4-day-old chicks. (b,d,e) Mean±s.e.m. (Kruskal–Wallis test and subsequent multiple comparisons, *P<0.05). (f) Mean±s.e.m. (U-test, *P<0.05). The number of animals used are indicated in each figure (b,d,e,f). DMSO, dimethylsulphoxide. Figure 4: T 3 acts as a determinant for the sensitive period. ( a ) The scheme for testing the effect of thyroid hormones for imprinting. ( b ) Dark-reared chicks were trained for imprinting with a yellow LEGO object and subsequently the preference for the yellow LEGO object was evaluated on a single day after hatching (from day 1 to day 10). The sensitive period closed on day 4 and chicks were not imprinted, whereas chicks injected with T 3 30 min before the training became imprintable from day 4 to day 6. ( c ) The scheme for testing the effect of thyroid hormones on 4-day-old chicks in d – f . Dark-reared chicks were trained for imprinting with a yellow LEGO object and the preference for the yellow LEGO object was evaluated on day 4 after hatching in the same way as shown in Fig. 2b . ( d ) Dose-dependent effects of thyroid hormones on 4-day-old chicks. ( e ) IMM injection of inhibitors (a thyroid hormone receptor antagonist, NH-3; a monocarboxylate transporter 8 inhibitor, BSP; Dio2 inhibitor, IOP) hampered the effect of thyroid hormones on 4-day-old chicks. ( f ) Effect of wortmannin on imprinting of 4-day-old chicks. ( b , d , e ) Mean±s.e.m. (Kruskal–Wallis test and subsequent multiple comparisons, * P <0.05). ( f ) Mean±s.e.m. ( U -test, * P <0.05). The number of animals used are indicated in each figure ( b , d , e , f ). DMSO, dimethylsulphoxide. Full size image Next we examined whether the mode of action of thyroid hormones in opening the sensitive period is a TR-mediated non-genomic action. IMM injection of NH-3 (ref. 24 ) or BSP hampered the effect of T 3 on 4-day-old animals, and IOP injection into the IMM eliminated the effect of T 4 ( Fig. 4e ), suggesting that T 3 converted from T 4 reopened a once closed sensitive period. Furthermore, wortmannin injection into the IMM 30 min before intravenous injection of T 3 hampered the effect of T 3 in 4-day-old animals ( Fig. 4f ), indicating that the action of thyroid hormone was short term, that is, a TR-mediated non-genomic action. The effects of exogenous T 3 in 4-day-old chicks Control experiments were performed. Chicks administered with norepinephrine, testosterone, caffeine, serotonin, or dopamine in the IMM did not demonstrate strong preference on day 4 after the sensitive period closed ( Fig. 5a ). In particular, drugs inducing arousal, activity, for example, caffeine, did not have the effect on chicks' preference that is seen with T 3 , indicating that T 3 has a specific role in imprinting and is not just producing a general effect of enhancing arousal, activity and so on. These results indicate that T 3 exhibits specific activity determining the start of the sensitive period. Exogenous T 3 injection 30 min before the imprinting training on day 4 after the sensitive period closed, light-exposed chicks showed the same strong preference for the yellow object as dark-reared chicks ( Fig. 5b ). These data indicate that T 3 as a sensitive period determinant enabled imprinting in chicks, regardless of whether they were reared in darkness or light. T 3 has an effect on the acquisition of memory during training, but does not directly affect preference during the test ( Fig. 5c ). The effect of exogenous T 3 on day 4 after the sensitive period had closed was mediated by the IMM region ( Fig. 5d,e ). 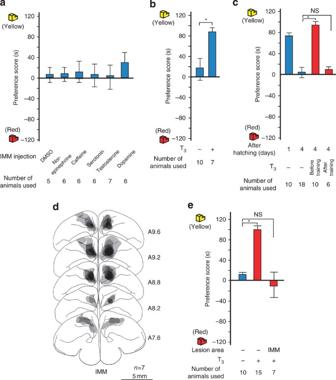Figure 5: The effects of exogenous T3on 4-day-old chicks. (a) Chicks administered with norepinephrine, caffeine, serotonin, testosterone or dopamine in the IMM as control reagents of thyroid hormones did not show strong preference on day 4. These reagents, including some neurotransmitters, a steroid hormone and a stimulant drug, did not induce strong preference after the sensitive period closed, suggesting that thyroid hormone exhibits specific activity determining the sensitive period. (b) In light-exposed chicks individually reared in separate cages, T3injection resulted in strong preference on day 4. The chicks were not able to see each other and kept in separate cages under light condition to prevent exposure to stimuli from moving objects. With exogenous T3injection 30 min before the imprinting training on day 4 after the sensitive period closed, light-exposed chicks showed the same strong preference for the yellow object as dark-reared chicks. (c) T3has an effect on the acquisition of memory during training but does not directly affect preference during the test. T3injected before the training allowed chicks to be imprinted on day 4, but T3injected after the training did not, suggesting that T3is effective on the acquisition of memory itself but not on the preference test score. (d,e) Effect of T3on imprinting on day 4 after the sensitive period closed was mediated by the IMM. (d) Histological reconstruction of ibotenic acid lesions in IMM. The lesioned areas are superimposed over coronal sections of telencephalon. (e) Bilateral lesion of IMM hampered the effects of injected T3on the acquisition of imprinting on day 4, whereas chicks without lesions could be imprinted with an injection of T3on day 4 after the sensitive period closed. (a,c,e) Mean±s.e.m. (Kruskal–Wallis test and subsequent multiple comparisons, *P<0.05). (b) Mean±s.e.m. (U-test, *P<0.05). (a,b,c,e) The training, testing and injection were performed following the experimental scheme shown inFig. 4c. The preference for the training object (yellow) was evaluated in the same way as shown inFig. 2b. The number of animals used are indicated in each figure (a,b,c,e). DMSO, dimethylsulphoxide; NS, nonsignificant. Figure 5: The effects of exogenous T 3 on 4-day-old chicks. ( a ) Chicks administered with norepinephrine, caffeine, serotonin, testosterone or dopamine in the IMM as control reagents of thyroid hormones did not show strong preference on day 4. These reagents, including some neurotransmitters, a steroid hormone and a stimulant drug, did not induce strong preference after the sensitive period closed, suggesting that thyroid hormone exhibits specific activity determining the sensitive period. ( b ) In light-exposed chicks individually reared in separate cages, T 3 injection resulted in strong preference on day 4. The chicks were not able to see each other and kept in separate cages under light condition to prevent exposure to stimuli from moving objects. With exogenous T 3 injection 30 min before the imprinting training on day 4 after the sensitive period closed, light-exposed chicks showed the same strong preference for the yellow object as dark-reared chicks. ( c ) T 3 has an effect on the acquisition of memory during training but does not directly affect preference during the test. T 3 injected before the training allowed chicks to be imprinted on day 4, but T 3 injected after the training did not, suggesting that T 3 is effective on the acquisition of memory itself but not on the preference test score. ( d , e ) Effect of T 3 on imprinting on day 4 after the sensitive period closed was mediated by the IMM. ( d ) Histological reconstruction of ibotenic acid lesions in IMM. The lesioned areas are superimposed over coronal sections of telencephalon. ( e ) Bilateral lesion of IMM hampered the effects of injected T 3 on the acquisition of imprinting on day 4, whereas chicks without lesions could be imprinted with an injection of T 3 on day 4 after the sensitive period closed. ( a , c , e ) Mean±s.e.m. (Kruskal–Wallis test and subsequent multiple comparisons, * P <0.05). ( b ) Mean±s.e.m. ( U -test, * P <0.05). ( a , b , c , e ) The training, testing and injection were performed following the experimental scheme shown in Fig. 4c . The preference for the training object (yellow) was evaluated in the same way as shown in Fig. 2b . The number of animals used are indicated in each figure ( a , b , c , e ). DMSO, dimethylsulphoxide; NS, nonsignificant. Full size image First imprinting primed the chicks for second imprinting Moreover, we found that chicks once imprinted on day 1 showed a higher capability to learn in subsequent training on day 4, indicating that the first imprinting primed the chicks for the second imprinting ( Fig. 6a,b ). The priming occurred irrespective of memory content (colour: Fig. 6a,b or shape: Fig. 6c,d ). The chicks did not forget the first object after learning the second object ( Fig. 6e ). Surprisingly, the potential to show preference was not blocked by IMM injection of NH-3 or intravenous injection of IOP just before training on day 4 ( Fig. 6b ). These findings suggest that the first increase in T 3 by imprinting training on day 1 was sufficient for chicks to acquire the potential to be imprinted at a later stage. In fact, T 3 concentration remained low when the imprinting training was done on day 4 ( Fig. 6f ). 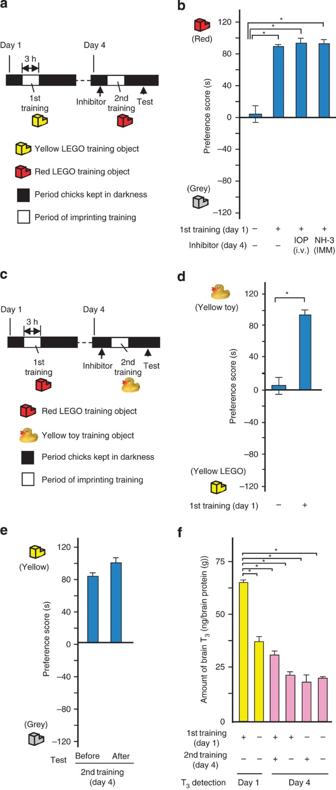Figure 6: Initial imprinting primed the chicks for second phase of imprinting. (a) The schemes to test the effect of initial imprinting for second phase of imprinting using objects of different colours. Chicks were trained with a yellow LEGO object on day 1. Then chicks were kept in darkness to prevent exposure to light. On day 4, the chicks were trained with a red LEGO object and the preference for the red LEGO object was evaluated 1 h later. (b) Chicks trained on day 1 became imprintable for the second training object (red LEGO object) on day 4, whereas dark-reared chicks could not be imprinted (n=10). The preference for the second training object was measured on day 4. The grey LEGO block was used as the control object in the simultaneous choice test. (c) The schemes to test the effect of first imprinting for second imprinting using the objects whose colour and shape were different. Chicks were trained with a red LEGO object on day 1. On day 4, the chicks were trained with a chick toy and the preference for the chick toy that was a different colour (yellow) and shape from the red LEGO object (first training object) was evaluated. (d) Chicks showed strong preference for the chick toy (second training object), but not for the control object (yellow) whose colour was the same as that of the chick toy (n=10). (e) The chicks were imprinted by a yellow LEGO object (first training object) on day 1 and remembered it well even after being imprinted by the red LEGO object (second training object) on day 4. The training and testing were performed following the experimental scheme shown ina. The preference for the first training object (yellow LEGO object) was measured before and after the second training. The grey LEGO block was used as the control object in the simultaneous choice test (n=10). (f) Chicks trained on day 4 (purple bars) show less brain T3than those trained on day 1 (yellow bar, leftn=6). (b,f) Mean±s.e.m. (Kruskal–Wallis test and subsequent multiple comparisons, *P<0.05). (d,e) Mean±s.e.m. (U-test, *P<0.05). Figure 6: Initial imprinting primed the chicks for second phase of imprinting. ( a ) The schemes to test the effect of initial imprinting for second phase of imprinting using objects of different colours. Chicks were trained with a yellow LEGO object on day 1. Then chicks were kept in darkness to prevent exposure to light. On day 4, the chicks were trained with a red LEGO object and the preference for the red LEGO object was evaluated 1 h later. ( b ) Chicks trained on day 1 became imprintable for the second training object (red LEGO object) on day 4, whereas dark-reared chicks could not be imprinted ( n =10). The preference for the second training object was measured on day 4. The grey LEGO block was used as the control object in the simultaneous choice test. ( c ) The schemes to test the effect of first imprinting for second imprinting using the objects whose colour and shape were different. Chicks were trained with a red LEGO object on day 1. On day 4, the chicks were trained with a chick toy and the preference for the chick toy that was a different colour (yellow) and shape from the red LEGO object (first training object) was evaluated. ( d ) Chicks showed strong preference for the chick toy (second training object), but not for the control object (yellow) whose colour was the same as that of the chick toy ( n =10). ( e ) The chicks were imprinted by a yellow LEGO object (first training object) on day 1 and remembered it well even after being imprinted by the red LEGO object (second training object) on day 4. The training and testing were performed following the experimental scheme shown in a . The preference for the first training object (yellow LEGO object) was measured before and after the second training. The grey LEGO block was used as the control object in the simultaneous choice test ( n =10). ( f ) Chicks trained on day 4 (purple bars) show less brain T 3 than those trained on day 1 (yellow bar, left n =6). ( b , f ) Mean±s.e.m. (Kruskal–Wallis test and subsequent multiple comparisons, * P <0.05). ( d , e ) Mean±s.e.m. ( U -test, * P <0.05). Full size image T 3 acts as a memory priming factor for learning As expected, the chicks treated with T 3 on day 1 were able to be imprinted on day 4 ( Fig. 7a,b ). This potential to show preference was not blocked by the IMM injection of NH-3 just before training on day 4 ( Fig. 7b ), indicating that the first increase in T 3 without visual experience on day 1 was sufficient to render chicks imprintable at a later stage. Furthermore, T 3 injection on day 1 enabled imprinting on day 8 ( Fig. 7c,d ), suggesting that injection of T 3 extends the sensitive period, and secondary learning can take place because the sensitive period remains open and closes later than without T 3 . We call this potential given by the wave of T 3 'memory priming' (MP). Even after the sensitive period closed, T 3 injection on day 4 enabled imprinting on day 8, while injection of T 3 before the imprinting training on day 8 did not ( Fig. 7e,f ), indicating that once MP is acquired, it continues to prime later learning, independent of visual experience. This led us to examine whether the first increase in T 3 could confer MP to learning other than imprinting. Chicks either injected with T 3 or trained for imprinting on day 1 showed a higher correct choice ratio in reinforcement learning of a colour discrimination pecking task on day 4 compared with those neither injected with T 3 nor trained for imprinting ( Fig. 7g,h ). This supports our idea that thyroid hormone confers MP and that MP which originates from imprinting may be followed by cascading layers of later learning. 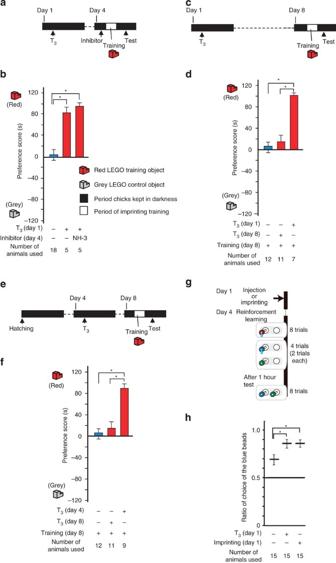Figure 7: T3acts as a memory priming factor for learning. (a,c,e,g) The schemes for experiments shown inb,d,f,h, respectively, to test the effect of MP for imprinting. (b,d,f) The preference for the red LEGO training object was evaluated using a grey LEGO object as the control in the simultaneous choice test. (a,b) Chicks intravenously injected with T3on day 1 became imprintable on day 4. The preference for the training object (red LEGO object) was measured on day 4. (c,d) Priming by T3injection on day 1 enabled imprinting on day 8. Chicks injected with T3on day 1 were kept in darkness until day 8. Then they were trained with a red LEGO object and the preference for the training object (red) was evaluated 1 h later. Memory priming keeps the sensitive period open for over 1 week. (e,f) Priming by T3injection even after the sensitive period closed enabled imprinting. After hatching, dark-reared chicks were injected with T3on day 4 when the sensitive period had closed. The chicks were kept in darkness until day 8 and then trained with a red LEGO object, and preference for the training object (red) was evaluated 1 h later. Even after the sensitive period closed, T3injection on day 4 enabled imprinting on day 8. (g,h) First increase of T3confers MP to learning other than imprinting. (g) The schemes to test the effect of MP for reinforcement learning of a colour discrimination pecking task. Chicks imprinted or injected with T3on day 1 were trained for reinforcement learning on day 4 and evaluated for correct choice ratio. (h) Effect of MP for reinforcement learning. (b,d,f,h) Mean±s.e.m. (Kruskal–Wallis test and subsequent multiple comparisons, *P<0.05). The number of animals used are indicated in each figure (b,d,f,h). Figure 7: T 3 acts as a memory priming factor for learning. ( a , c , e , g ) The schemes for experiments shown in b , d , f , h , respectively, to test the effect of MP for imprinting. ( b , d , f ) The preference for the red LEGO training object was evaluated using a grey LEGO object as the control in the simultaneous choice test. ( a , b ) Chicks intravenously injected with T 3 on day 1 became imprintable on day 4. The preference for the training object (red LEGO object) was measured on day 4. ( c , d ) Priming by T 3 injection on day 1 enabled imprinting on day 8. Chicks injected with T 3 on day 1 were kept in darkness until day 8. Then they were trained with a red LEGO object and the preference for the training object (red) was evaluated 1 h later. Memory priming keeps the sensitive period open for over 1 week. ( e , f ) Priming by T 3 injection even after the sensitive period closed enabled imprinting. After hatching, dark-reared chicks were injected with T 3 on day 4 when the sensitive period had closed. The chicks were kept in darkness until day 8 and then trained with a red LEGO object, and preference for the training object (red) was evaluated 1 h later. Even after the sensitive period closed, T 3 injection on day 4 enabled imprinting on day 8. ( g , h ) First increase of T 3 confers MP to learning other than imprinting. ( g ) The schemes to test the effect of MP for reinforcement learning of a colour discrimination pecking task. Chicks imprinted or injected with T 3 on day 1 were trained for reinforcement learning on day 4 and evaluated for correct choice ratio. ( h ) Effect of MP for reinforcement learning. ( b , d , f , h ) Mean±s.e.m. (Kruskal–Wallis test and subsequent multiple comparisons, * P <0.05). The number of animals used are indicated in each figure ( b , d , f , h ). Full size image Learning that occurs during the sensitive period lays the foundation for future learning in some cases [6] . A number of features are common to imprinting and visual cortical plasticity [31] . Visual cortical plasticity has been studied since its discovery by Hubel and Wiesel [32] using cats. Sensitivity to monocular deprivation is restricted to a sensitive period after eyes open. The onset of plasticity can be delayed by directly preventing the maturation of GABA-mediated transmission in the visual cortex [33] , suggesting that the sensitive period depends on the proper level of inhibitory transmission. Therefore, it might be interesting to study the relationship between thyroid hormone signalling and GABA transmission in chicks' imprinting. Visual cortical plasticity in mice comes to an end when further maturation of the neuronal network is inhibited by myelination [34] , [35] . In chicks' imprinting, myelination may consolidate the neural circuit and suppress the T 3 effect, limiting the synaptic plasticity in the opening of the sensitive period for imprinting. According to the synaptic tagging and capture hypothesis [36] , strong tetanization of one synaptic pathway leads to local tag setting and synthesis of diffusible plasticity-related proteins. The plasticity-related proteins are then captured by tagged synapses and the resulting complex is necessary for the maintenance of late long-term potentiation. Other molecular events like synaptic tagging and capture downstream of T 3 may trigger lasting changes in synapses expressing plasticity in chicks' imprinting, and significant modification may occur in the structure of synapses. Thyroid hormone has been shown to have a critical role in differentiation, growth and metabolism [23] . For example, T 3 deficiency during brain development in humans has been reported to be associated with irreversible mental disability and profound neurological disorder, including impairment of learning and memory [27] . In this case, T 3 is considered to function through genomic action with regard to the mode of action of T 3 . However, in imprinting, T 3 binds to TR in the cytoplasm of neuronal cells, and the resulting heterodimer may lead to subsequent changes in neurons through non-genomic action in vivo . This is one of the features that distinguish T 3 effect in imprinting from the well-known T 3 function on neonatal brain development through genomic action. In this study, we show that the thyroid hormone signalling is upregulated in broad areas of chick brain including the IMM, the area responsible for imprinting, suggesting that acute thyroid hormone signalling may be involved in a variety of brain functions around the time of hatching. However, when we conducted a control experiment injecting T 3 in a more apical region than the IMM, T 3 had no effect on the chicks' preference, suggesting that T 3 effect on the IMM is specific. In the course of imprinting, the wave of T 3 beyond a certain threshold concentration likely confers MP through rapid non-genomic action in the course of visual imprinting training. On the other hand, 4 days after hatching, T 3 levels decreased to background level at the same time that dark-reared chicks should no longer be able to be imprinted, but exogenous T 3 enabled the imprinting. The exogenous T 3 on day 4 seems to confer MP, probably through mainly non-genomic action ( Fig. 8 ). 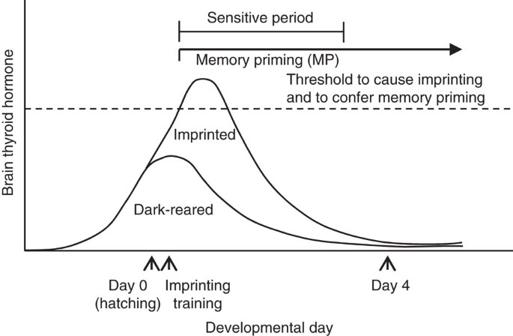Figure 8: T3is a determinant for the sensitive period and primes later learning. The main findings of our paper are summarized in the schematic. The concentration of 3,5,3′-triiodothyronine (T3) in brains peaked around hatching, and further increase of T3induced by imprinting was required for imprinting. On day 4, T3concentration remained low even after imprinting training and chicks could no longer be imprinted. This is why the sensitive period is normally restricted to the first 3 days. However, in our study, 4 days after hatching, in non-imprinted chicks whose sensitive period had closed, exogenous T3was able to reopen it and enable imprinting. Thus, T3is a determining factor for the start of the sensitive period of imprinting. Moreover, the additional wave of T3induced in the course of imprinting appears to confer memory priming (MP) through rapid non-genomic action. Once chicks are primed and conferred MP, the sensitive period remains open for over 1 week, driving subsequent learning and enhancing memory. Even after the sensitive period closed without the first additional wave of T3induced by imprinting, exogenous T3was able to confer MP mainly through acute non-genomic action. Figure 8: T 3 is a determinant for the sensitive period and primes later learning. The main findings of our paper are summarized in the schematic. The concentration of 3,5,3′-triiodothyronine (T 3 ) in brains peaked around hatching, and further increase of T 3 induced by imprinting was required for imprinting. On day 4, T 3 concentration remained low even after imprinting training and chicks could no longer be imprinted. This is why the sensitive period is normally restricted to the first 3 days. However, in our study, 4 days after hatching, in non-imprinted chicks whose sensitive period had closed, exogenous T 3 was able to reopen it and enable imprinting. Thus, T 3 is a determining factor for the start of the sensitive period of imprinting. Moreover, the additional wave of T 3 induced in the course of imprinting appears to confer memory priming (MP) through rapid non-genomic action. Once chicks are primed and conferred MP, the sensitive period remains open for over 1 week, driving subsequent learning and enhancing memory. Even after the sensitive period closed without the first additional wave of T 3 induced by imprinting, exogenous T 3 was able to confer MP mainly through acute non-genomic action. Full size image Metaplasticity is a proposed paradigm in which the first stimulation of activity (priming) changes the electrophysiological state of neurons or synapses, a change which persists until a second stimulus of activity induces long-term potentiation or long-term depression [37] . This feature distinguishes metaplasticity from the conventional form of plasticity modulation in which the modulating and regulated events overlap in time. The relationship between learning and metaplasticity is unclear [37] , but we found that the first increase in T 3 acts as a priming factor and confers MP to allow chicks to gain the potential to be imprinted at a later stage, while dark-reared animals cannot be imprinted at all. Thus, we assume MP to be a good example of metaplasticity in vivo and that MP is maintained for long periods once animals have achieved that state. Some cases of hormonal factors influencing the sensitive period of imprinting have been reported [10] , [11] , [12] . A rise in the corticosterone levels in ducklings was assumed to define the end of the sensitive period. However, corticosterone turned out to indirectly influence the sensitive period, followed by inhibition of the subsequent reaction [10] . It is noteworthy that T 3 can open a once closed sensitive period in chicks and enable imprinting once again. This suggests that the beginning of the sensitive period in imprinting may be regulated by a simple hormonal level. In a manner similar to that proposed in electrophysiological research [37] , the priming activity of T 3 may trigger lasting changes in synapses to express plasticity in chicks' imprinting, and there may be significant modulation in the structure of dendritic spines as a result of priming. It has been reported that the neuronal circuits can be rapidly and persistently modified by certain forms of learning [38] . The functional relationship between dendritic spine remodelling and the priming by T 3 remains to be elucidated. Predispositions refer to intrinsic perceptual preferences that develop in young animals without visual experience with the particular stimuli involved [39] . It has been reported that the filial predisposition emerges in dark-reared chicks given some nonspecific experience for 2–24 h during a sensitive period without imprinting training [40] . The predisposition is suggested to bias imprinting before chicks learn the characteristics of individuals [40] . The neural substrate for the predisposition is located outside the IMM [41] . As we showed in this report, MP is likely to have some different characteristics from such predisposition, although MP and the predisposition emerge in dark-reared chicks, and visual experience is not required for their expression. MP by T 3 occurs within 30 min through specific TR signalling in chicks, regardless of whether they were reared in darkness or light, and the IMM is required for the expression of MP. In addition, predisposition is expressed as enhancement of training-independent intrinsic preference, but MP can elicit robust preference in learning acquired through training, although the possibility that MP utilizes some features of predisposition for expression cannot be excluded. We propose that imprinting, serving as a primer, is crucial to the chick's learning process. Our data provide evidence that thyroid hormone confers MP and that MP which originates from imprinting may be followed by cascading layers of later learning. The idea that one learning process could be based on another has been proposed [42] . In sexual imprinting, the imprinting process has been assumed to cause the 'consumption' of a limited amount of memory space illustrated using the model of a set of empty boxes filled with balls [43] . However, the feature of the primer is difficult to incorporate in this model. We instead propose a 'champagne tower' model. In this model, MP as well as T 3 has certain threshold levels. Champagne glasses (each representing learning with a sensitive period) are arranged in a pyramid, and champagne (flow of MP formed by a hormone) is poured into the top glass (imprinting, early learning) until it overflows and trickles down into the lower layers of glasses (later learning). When the champagne does not flow fully into each glass within a limited time, the sensitive period ends. However, if the champagne level exceeds the top of the glass, the overflow pours down to the next layer of glasses (later learning). In conclusion, our results imply that MP occurs depending on necessity in the early development of each animal species and is key to learning at a later time. Imprinting is an example of early learning accompanied by MP mediated by the hormone T 3 ( Fig. 8 ). We believe MP to be an expression of the neural circuit to start the sensitive period to ensure the acquisition and maintenance of learning. Priming does not necessarily include sensory information, and once animals have achieved priming, the sensitive period starts and remains open. MP is an endogenous system that can be separated from experience at the molecular level. In the case of imprinting, MP is conferred simultaneously with experience. We assume that once MP is achieved, it is maintained for long periods. It is possible that the sensitive period closes only if MP is not conferred at an appropriate time of development. Under natural conditions, animals will learn spontaneously with the help of parents and siblings. In a sense, the closing of the sensitive period for learning may not exist under usual physiological conditions probably because the sensitive period does not close as long as MP is acquired. Therefore, the term, 'sensitive period' or 'critical period' in our study may be linked to priming as well as learning. That is, the sensitive period for MP can be estimated to be about 6 days after hatching in the imprinting of chicks ( Fig. 4b ). There may exist determining factors among higher intelligent animals as well that can cause the opening of a sensitive period. The implications of this study reach beyond the sensitive period of imprinting and learning in chicks and deepen our understanding of the processes of learning. Animals The experiments were conducted under the guidelines of the committee on animal experiments of Teikyo University. Newly hatched domestic chicks of the Cobb strain ( Gallus gallus domesticus ) were used. Fertilized eggs were obtained from a local supplier (3-M, Nagoya, Japan). After hatching, the chicks were placed in darkness to prevent exposure to light until they were subjected to the imprinting training [44] . The chicks were given water from day 3 and they ate voluntarily even in darkness. The locomotor activity and colour discrimination ability of the dark-reared chicks were the equivalent of those of the chicks reared in separate cages under light condition. Chicks kept in darkness for 8 days after hatching were able subsequently to form a strong preference for an object by T 3 injection on day 1 and continued living in good health. Detection of the conversion of T 4 from T 3 in brain 125 I-labelled T 4 was injected intravenously (about 4×10 6 c.p.m., 2,200 Ci mmol −1 , PerkinElmer) into chicks, which were kept in dark plastic enclosures for 1 h. Then brain and blood samples were collected under deep anaesthesia. Brain thyroid hormones were extracted with methanol/chloroform as described [45] . 125 I-labelled thyroid hormones were immunoprecipitated using an excessive amount of rabbit anti-T 3 antibody (Sigma-Aldrich, T2777) or rabbit anti-T 4 antibody (Sigma-Aldrich, T2652), and the radioactivities of the precipitates were counted by gamma counter. Adding serially diluted 125 I-labelled thyroid hormones to brain extract or serum, we confirmed that 125 I-labelled thyroid hormones were precipitated by an excessive amount of antibodies in a dose-dependent manner. Then we calculated the ratio of 125 I-labelled T 3 to T 4 of the precipitated fractions in brain extract or serum. Each brain extract or serum was added in duplicate to 0.075 M barbital buffer (pH 8.6) containing 0.1% gelatin, 0.15% bovine γ-globlin (Sigma-Aldrich), 8-anilino-1-naphthalene sulphonic acid. The anti-T 3 antibody or the rabbit anti-T 4 antibody was added to a final dilution of 1:1,250. They were incubated for 2 h on ice, then precipitated by addition of cold polyethylene glycol 6000 (Sigma-Aldrich). After incubated for 30 min on ice, the samples were centrifuged at 3,000 r.p.m. for 30 min at 4 °C. The supernatant was aspirated and the radioactivity of the precipitates counted by gamma counter. IOP was injected 1 h before the injection of 125 I-labelled T 4 . 125 I-labelled T3 and 125 I-labelled T4 were obtained from PerkinElmer. Intravenous injection of thyroid hormones and inhibitors IOP (1 mM, Tokyo Chemical Industry) was dissolved in 0.05 M NaOH and rebuffered to pH 7.4 by 0.2 M HCl. Phloretin (Calbiochem) was dissolved in ethanol (200 mM) then diluted in PBS to a final concentration of 1 mM. A volume of 100 μl of each inhibitor solution was injected intravenously. T 3 or T 4 (10 μM, Sigma-Aldrich) was dissolved in 0.002 M NaOH and 0.9% NaCl. Twenty hours after hatching, T 3 or T 4 was injected intravenously and the resulting concentration of T 3 or T 4 in serum was ~20 ng ml −1 . In our experiments, the concentrations of T 3 and T 4 in serum were calculated within a time period of ~30 min between the intravenous injections and imprinting training. The difference in half-life between T 3 and T 4 did not affect the measurements so much under our acute experimental conditions because the half-lives of chick T 3 and T 4 have been reported to be 1.5 and 1.2 h, respectively [46] . Control vehicle was injected intravenously in each experiment. Imprinting training was initiated 30 min after the injection. In vivo injection into the IMM region The injection was performed as described [47] with modifications. Chicks were fixed on a stereotaxic apparatus under 2% isofluorane/air mixture. The skin over the skull surface was incised, and a small piece (0.1 mm×0.1 mm) of the dura matter was cut to expose the telencephalon. Stereotaxic coordinates for the IMM were as follows: 2.9 mm anterior to the bregma, 1.3 mm lateral to the midline and 2.0 mm in depth. All the inhibitors or reagents were dissolved in dimethylsulphoxide. IOP (100 μM), BSP (100 μM, Sigma-Aldrich), NH-3 (10 μM), wortmannin (10 μM, Wako), norepinephrine (10 μM, Sigma-Aldrich), testosterone enanthate (10 μM, Wako), caffeine (10 μM, Sigma-Aldrich), serotonin (10 μM, Sigma-Aldrich) and dopamine (10 μM, Sigma-Aldrich) or T 3 (10 μM) were injected at a rate of 14 nl min −1 for 35 min using an automatic injector (Nanoject II, Drummond). The resulting amount of T 3 in brains was about 30 ng per brain proteins (g). Control vehicle was injected into the IMM in each experiment. Chicks were returned to the dark breeder to recover from the anaesthesia for 30 min, then subjected to the training for imprinting. Behavioural training and testing Training for imprinting was carried out by the method of Izawa et al . [44] with modification. A training chamber equipped with a computer-controlled rubber belt (8 cm wide, 43 cm long, 15 cm high) and an infrared sensor was used for the training for imprinting. A microcomputer (RCX2.0, Robotics Invention System, LEGO Co., Tokyo, Japan) commanded the running belt to move backward when a chick broke the beam of an infrared sensor. The training object (a yellow LEGO block, 4.7 × 6.2 cm, 5.0 cm high) was placed 20 cm in front of the infrared sensor and illuminated from above by a 100 W fiber optic light. Training typically started about 18 h after hatching. Before training started, chicks were kept in a dark breeder. Each chick was exposed to the training object in two 1-h training sessions separated by a 1-hour interval. Each training session consisted of 12 successive runs (4 min each) at 1-min intervals. In each run, the object was rotated six times for 30 s, with 10-sec pauses in between. During the 30-sec movement period, the object continuously repeated clockwise and anticlockwise rotations (~25°) every 0.5 s. In this training, we used only visual imprinting stimuli and no auditory stimuli. During the 1-min inter-run intervals, the illumination was turned off and the chick was left in darkness. During the 1-hour inter-session interval, the chick was returned to the dark breeder. Testing for imprinting was also carried out by the method of Izawa et al . [44] with modification. After completion of the training session, to measure the strength of chick's preference for the training object, simultaneous choice test was performed using a T-maze with the main alley 20 cm long, 8 cm wide and 15 cm high, and the side arm 69 cm long ( Fig. 2b; Supplementary Movie 1 ). At the end of each side arm, the training object (the yellow LEGO block) or a novel control object (a red LEGO block) was placed and programmed to rotate synchronously according to the same schedule as in the training. A chick starts from the main alley, is allowed to walk freely and choose and approach one of the objects. Except for the time chicks stayed in the approach areas, they spent time in the intermediate area between the two approach areas. The test apparatus interior was illuminated by a 100 W fiber optic light (LG-PS2, Olympus, Tokyo, Japan). During 120 s, we measured the total time the chick spent in each approach area near the objects at the end of each side arm (13 cm long). Preference for the training object (yellow) was measured by the difference in approach time; the total time a chick spent near the control object (red) was subtracted from the total time the chick spent near the training object (yellow). The two values usually totalled ~90 s and <120 s. The remaining 30 s is accounted for by the time the chicks spent in the intermediate area between compartments. The average of preference scores derived from four successive trials is used as the individual chick's preference score. For MP, chicks were trained with a yellow LEGO object or injected with T 3 on day 1. Then chicks were kept in darkness to prevent exposure to light. On day 4, the chicks were trained with a red LEGO object, and the preference for the red LEGO object was evaluated 1 h later. A grey LEGO block was used as the control object in the simultaneous choice test. Inhibitors were injected 30 min before initiation of training on day 4. Typical time lines of the behavioural experiments testing the effect of MP are shown in the figures. Experimental conditions varied by experiment (See details in each corresponding Figure legend.). Reinforcement learning of a colour discrimination pecking task was performed as described previously [44] . The chick was initially trained to associate pecking a bead with a drop of water. A brown bead was presented through one of a pair of holes. If the chick pecked the bead, a drop of water was given. The hole through which the bead was presented was alternated. Then the chick was trained to associate a blue bead with a drop of water. When a green bead was presented, water was not given. Of the blue and green beads each colour was presented only twice. To test the effect of MP for reinforcement learning, chicks that were trained for imprinting or injected with T 3 on day 1 were trained for reinforcement learning and evaluated for correct choice ratio on day 4. Methods for microarray analysis, quantitative reverse transcription–polymerase chain reaction, radioimmunoassay, IMM lesions, immunohistochemistry, western and northern blotting, in situ hybridization, and cDNA cloning of Dio2 are described in the Supplementary Methods . Accession codes: All raw and normalized data obtained from cDNA microarray analysis have been deposited in the Gene Expression Omnibus (GEO; accession code: GSE31055 ). How to cite this article: Yamaguchi, S. et al . Thyroid hormone determines the start of the sensitive period of imprinting and primes later learning. Nat. Commun. 3:1081 doi: 10.1038/ncomms2088 (2012).